Two sequential cleavage reactions on cruciform DNA structures cause palindrome-mediated chromosomal translocations Gross chromosomal rearrangements (GCRs), such as translocations, deletions or inversions, are often generated by illegitimate repair between two DNA breakages at regions with nucleotide sequences that might potentially adopt a non-B DNA conformation. We previously established a plasmid-based model system that recapitulates palindrome-mediated recurrent chromosomal translocations in humans, and demonstrated that cruciform DNA conformation is required for the translocation-like rearrangements. Here we show that two sequential reactions that cleave the cruciform structures give rise to the translocation: GEN1-mediated resolution that cleaves diagonally at the four-way junction of the cruciform and Artemis-mediated opening of the subsequently formed hairpin ends. Indeed, translocation products in human sperm reveal the remnants of this two-step mechanism. These two intrinsic pathways that normally fulfil vital functions independently, Holliday-junction resolution in homologous recombination and coding joint formation in rearrangement of antigen-receptor genes, act upon the unusual DNA conformation in concert and lead to a subset of recurrent GCRs in humans. Gross chromosomal rearrangement (GCR) is generally acknowledged to be generated by DNA breaks at two different chromosomal loci followed by illegitimate repair of these broken ends. Although DNA breakage by ionizing radiation or reactive oxygen species takes place accidentally and the breakpoints are distributed in a random fashion, certain chromosomal regions are susceptible to DNA breakage manifesting as hotspots for GCR breakpoints. The most frequent recurrent GCR in humans is the Robertsonian translocation with a high de novo mutation rate of ~3.9 × 10 −4 , and it takes place between highly repetitive tandem sequences at the centromeric regions [1] . Inverted repeats or palindromic sequences are also hotspots for breakpoints of GCRs, because intra-strand annealing of the palindromic DNA potentially forms single-stranded hairpin or double-stranded cruciform structures. There are two main hypotheses for the genomic instability of the palindrome. The palindromic DNA may adopt a hairpin structure in the long single-stranded DNA of the lagging-strand template that may serve as a replication barrier [2] . Replication stalling may induce replication slippage or template switching, leading to deletions or duplications of the nearby genomic region [3] , [4] . In addition, inverted repeats often trigger dicentric or acentric chromosome formation, possibly caused by template switching upon replication resumption after a pausing at the inverted repeats [5] . In sharp contrast, another hypothesis is that a structure-specific endonuclease might cleave the secondary structure formed by the palindrome, leading to frequent DNA breakage [6] , [7] . A subset of recurrent constitutional chromosomal translocations in humans develops between two palindromic AT-rich repeats (PATRRs) at different chromosomal loci that share no sequence homology [8] . One of the best-characterized constitutional translocations is the recurrent t (11;22)(q23;q11.2), carriers of which are often identified after a birth of offspring manifesting supernumerary-der(22) t (11;22) syndrome (Emanuel syndrome: accession code OMIM no. 609029). All of the constitutional t (11;22)s develop between two PATRRs on chromosomes 11 and 22 that consist of only several hundreds base pairs [9] , [10] . In addition, de novo t (11;22)s (1.0–0.1 × 10 −4 ) are found in sperm from healthy males [11] . The PATRRs manifest size polymorphisms, and the symmetry and length of the PATRRs greatly influence the de novo translocation frequency [12] , [13] . Thus, we proposed that the palindromic sequences form a cruciform conformation in vivo , and this conformation could induce DNA breakage that results in illegitimate joining, leading to a reciprocal translocation. To date, more than five other translocation-associated PATRRs have been identified, suggesting that palindrome-mediated chromosomal translocations are one of the important pathways generating GCRs in humans [14] , [15] , [16] , [17] , [18] . We have previously reported a model system for PATRR-mediated translocations using two plasmids containing either PATRR11 or 22 (ref. 19 ). When the plasmids were introduced into a human cell, they produced rearranged molecules that have junction sequence with features similar to those of human t (11;22)s [20] , [21] . The translocation-like rearrangements in this model system were observed only when both PATRRs extruded cruciform structures. Because the introduced plasmids carry a non-replicating plasmid backbone, the results suggest that some intrinsic structure-specific nucleases may recognize the secondary structures and cleave the PATRR at the centre, which is followed by repair via the non-homologous end-joining (NHEJ) pathway. In contrast, endogenous PATRRs on the host chromosomes never generate translocations in somatic cell lines [22] . The model system implies that human somatic cells may have the molecular machinery that can perform the process of PATRR-mediated chromosomal translocations, with the exception of the initial step, cruciform formation at the PATRRs. Two distinct hypotheses of the cleavage manner for cruciform DNA in vivo have been proposed: centre break and diagonal cleavage ( Fig. 1a ) [23] , [24] , [25] . The fact that translocation breakpoints cluster at the centre of the palindrome leads directly to the centre-break hypothesis: breakage at the two cruciform apices. The other hypothesis, diagonal cleavage or resolution, was previously proposed as an intermediate product in the rearrangement of yeast chromosomes harbouring a palindromic sequence [7] . In this report, we attempt to identify the molecular pathway that leads to palindrome-mediated translocation in humans by screening candidate genes using the small interfering RNA (siRNA) technique in our translocation model system. 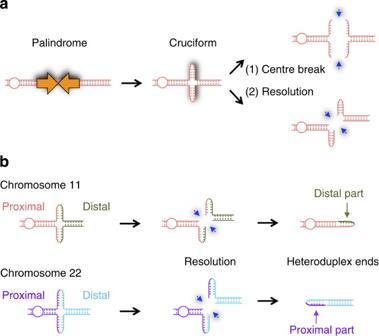Figure 1: Two distinct way of cruciform cleavagein vivo. (a) Two hypotheses for the mechanism of cruciform cleavage: centre-break and cruciform resolution. (b) The resolution of the cruciform produces heteroduplex DNA in the newly formed hairpin ends, which consist of proximal and distal units of the palindromes. Nucleotide differences between the proximal and distal arms can be utilized to discriminate the origins of the arms. Exchange between proximal and distal arms indicates the signature of the heteroduplex. Figure 1: Two distinct way of cruciform cleavage in vivo . ( a ) Two hypotheses for the mechanism of cruciform cleavage: centre-break and cruciform resolution. ( b ) The resolution of the cruciform produces heteroduplex DNA in the newly formed hairpin ends, which consist of proximal and distal units of the palindromes. Nucleotide differences between the proximal and distal arms can be utilized to discriminate the origins of the arms. Exchange between proximal and distal arms indicates the signature of the heteroduplex. Full size image Sequence of the rearrangement junction evokes cruciform resolution Our previous report demonstrated that two PATRR sequences induced a translocation-like rearrangement reaction in human cultured cells only when both PATRRs extruded cruciform structures [19] . To investigate how the cruciform was cleaved and illegitimately joined, we first analysed the junction sequences of the rearranged molecules in the model system using translocation-specific PCR with a primer flanking the proximal side of PATRR11 and one flanking the distal side of PATRR22. Sequence analysis of the cloned junction products revealed that breakpoints were heterogeneous but consistently located at the centre of the palindrome. The two fragments were joined with either no or limited microhomology, typically accompanied by deletion of several nucleotides at the breakpoints [19] . Each of the PATRR11 and 22s introduced into plasmids have nucleotide differences at several sites between their proximal and distal arms. We determined a pattern of three different nucleotides that allow discrimination between the proximal and distal arms of PATRR11 in 40 junction clones. Because junction PCR was carried out with a primer flanking the proximal side of PATRR11 and one flanking the distal side of PATRR22, a junction should be identified as a fusion of the proximal arm of PATRR11 and the distal arm of PATRR22. However, when the three nucleotide positions of PATRR11 were examined, only 15 of the 40 junctions showed proximal sequence at all three of the positions ( Table 1 ). Another 17 junctions showed proximal-to-distal nucleotide conversion at all of the positions. The remainder displayed a mixed pattern of conversion. Similar results were obtained at two-nucleotide positions of PATRR22 ( Supplementary Table S1 ). Each of these conversions of PATRR11 and 22 were found independently in 40 junction clones. This phenomenon cannot be explained by a simple ‘centre-break mechanism’ as has been proposed for palindrome-mediated rearrangement. We speculate that the PATRR is cut diagonally at the four-way junction of the cruciform structure ( Fig. 1a ). In this scenario, a diagonal cut produces hairpin-capped DNAs that create a heteroduplex consisting of a proximal arm for one strand and a distal arm for the other strand ( Fig. 1b ). The resulting hairpin-ended DNA should carry several sequence mismatches in the duplex DNA, which may potentially be repaired using one of the strands as template at a later step. Table 1 Three nucleotide changes of the PATRR11 in the junction sequences Full size table We attempted to find evidence for such heteroduplex DNA in the rearranged products obtained in this model system. When template DNA was diluted before translocation-specific PCR to amplify the junction molecule from a single molecule per tube, all of the junction sequences demonstrated a single sequence pattern either of proximal or distal sequence at each of the three distinguishable positions. However, when a mismatch repair (MMR) protein MSH2 was knocked down using siRNA, 2 junction products out of 19 showed a mixture of proximal and distal PATRR11 sequences at the three positions ( Supplementary Fig. S1a,b,c ). This indicated that the template DNA included heteroduplex DNA that should have been repaired by the MMR system into either proximal or distal sequence. Similarly, 1 out of 14 junctions showed mixture of proximal and distal PATRR22 sequences at the two distinguishable positions ( Supplementary Fig. S1b,c ). The presence of the heteroduplex structure suggests that the cruciform DNA at the PATRR is initially cleaved diagonally at the four-way junction. Diagonal digestion of the cruciform in the first cleavage Next, we carried out Southern blot analysis to demonstrate the diagonal cleavage of the four-way junction of the cruciform suggested by sequence analysis. The PATRR22 plasmid with its extruded cruciform was introduced into HEK 293 cells. To monitor cleavage, plasmids were collected at different time points and digested with a restriction enzyme ( Supplementary Fig. S2a ). A 1.3-kb band, derived from plasmid cleaved at the PATRR, appeared 30 min after transfection ( Fig. 2a , left), The intensity of the band continued to increase until 3 h after transfection. This cleavage was a cruciform-specific reaction ( Fig. 2a , lanes 7 and 8). 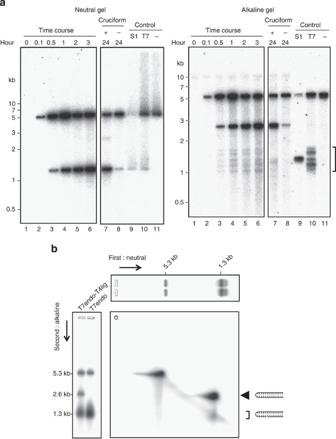Figure 2: DNA breakage of the PATRR via diagonal cleavage of cruciform DNA. (a) Southern blot analysis for the distal side of PATRR22 in native (left) and alkaline (right) conditions. Schematic representation of the analysis was shown inSupplementary Fig. S1a. Plasmids prepared by the alkaline-SDS method were used for a time-course analysis (0.1–24 h). In addition, plasmids obtained by the Triton method incubated in low-ionic conditions (lane 7) or those with topoisomerase I treatment (lane 8) were also used for the transfection. As size controls, cruciform-extruded PATRR22 plasmid DNAs with S1 nuclease (S1) or T7 endonuclease I (T7) treatment, or without any treatment (–), were used. The main band at 1.3 kb under neutral conditions (left panel) and at 2.6 kb under alkaline conditions (right panel) indicate closed hairpin formation at the PATRR-cleavage site. Lower bands at the 1–1.6 kb interval (bracket) are possibly derived from hairpin ends with un-repaired nicks. (b) Two-dimensional gel electrophoresis. The sample obtained 6-h after transfection was electrophoresed horizontally in native conditions and then vertically in alkaline conditions. As a size control, T7 endonuclease I-digested DNAs (T7endo) or that which was followed by T4 DNA ligase reaction (T7endo-T4Lig) were used. The results of one-dimensional gel electrophoresis of the size controls were superimposed on the two-dimensional gel image. An arrowhead indicates the closed hairpin-ended fragment, which is equivalent to a 2.6-kb band of the control sample treated with T4 DNA ligase. Figure 2: DNA breakage of the PATRR via diagonal cleavage of cruciform DNA. ( a ) Southern blot analysis for the distal side of PATRR22 in native (left) and alkaline (right) conditions. Schematic representation of the analysis was shown in Supplementary Fig. S1a . Plasmids prepared by the alkaline-SDS method were used for a time-course analysis (0.1–24 h). In addition, plasmids obtained by the Triton method incubated in low-ionic conditions (lane 7) or those with topoisomerase I treatment (lane 8) were also used for the transfection. As size controls, cruciform-extruded PATRR22 plasmid DNAs with S1 nuclease (S1) or T7 endonuclease I (T7) treatment, or without any treatment (–), were used. The main band at 1.3 kb under neutral conditions (left panel) and at 2.6 kb under alkaline conditions (right panel) indicate closed hairpin formation at the PATRR-cleavage site. Lower bands at the 1–1.6 kb interval (bracket) are possibly derived from hairpin ends with un-repaired nicks. ( b ) Two-dimensional gel electrophoresis. The sample obtained 6-h after transfection was electrophoresed horizontally in native conditions and then vertically in alkaline conditions. As a size control, T7 endonuclease I-digested DNAs (T7endo) or that which was followed by T4 DNA ligase reaction (T7endo-T4Lig) were used. The results of one-dimensional gel electrophoresis of the size controls were superimposed on the two-dimensional gel image. An arrowhead indicates the closed hairpin-ended fragment, which is equivalent to a 2.6-kb band of the control sample treated with T4 DNA ligase. Full size image We further carried out electrophoresis in a denaturing alkaline gel followed by Southern blotting. A major cleaved band is seen at 2.6 kb, which is twice of the size of what is observed in a neutral gel ( Fig. 2a , right). These results suggest that the cleaved DNA end forms a closed hairpin. Because the hairpin ends cannot be produced by centre breakage of the cruciform, it is likely that the PATRR22 plasmids are cut by diagonal cleavage, resolving the cruciform structure. Indeed, the presence of hairpin-capped DNA was confirmed by Southern blotting of a two-dimensional gel ( Fig. 2b ). The hairpin-capped DNAs were also present at the other end of the cleaved PATRR22, supporting diagonal cleavage at the four-way junction ( Supplementary Fig. S2b , left). Similar result was obtained with PATRR11 plasmid ( Supplementary Fig. S2b , right). Because diagonal cleavage at the four-way junction of the cruciform is predicted to generate a pair of hairpin ends with nicks at the cleaved sites, it is possible that the closed hairpin ends detected in the Southern blots could be generated by sealing the nicks with an endogenous ligase activity. In addition, some minor bands were also observed between 1.0 and 1.6 kb, possibly originating from intermediate products that were left unsealed at the nicks ( Fig. 2a (right) ). To confirm resolution of the cruciform at the four-way junction, the cleavage site within the PATRR was determined at the nucleotide level. A ligation-mediated PCR was carried out to map the 5′ end of these intermediate products before the sealing of the nicks. In an analysis of the proximal end of PATRR11, an approximately 550 bp product appeared in the sample obtained 0.5 h after transfection, which was increased in amount in the 6-h sample ( Fig. 3a , arrowhead). The size of the product was 180 bp longer than that of the product from a sample treated with S1 nuclease, which is expected to cut at the palindromic centres (lane 6). This indicates that the 5′ end of the proximal breakpoint was located about 180 bp proximal to the centre of the palindrome. The distal end was also mapped about 180 bp distal to the centre. Sequencing of the products confirmed the symmetric cuts on each strand, which strongly suggest diagonal cleavage of the four-way junction of the cruciform. This likely occurs by introduction of two nicks, one near the proximal end of the PATRR in the top strand and the other near the distal end of the bottom strand of the cruciform ( Fig. 3c ). The directional preference of diagonal cleavage is similar to that of four-way junction activity such as T4 endonuclease VII and T7 endonuclease I in resolution of cruciform-extruding plasmids [26] , [27] . Analysis of the PATRR22 revealed similar symmetric nicks about 110 bp away from the centre ( Fig. 3b ). Taken together, it appears that both PATRR11 and 22 are cut diagonally at the four-way junction of the cruciform, and that most of the cleaved ends undergo nick repair to form closed hairpin-capped DNA ends. We note that sequence of the cleavage site within the PATRR by ligation-mediated PCR provided no evidence for products with a proximal-to-distal exchange (data not shown). This suggests that the proximal-to-distal change take place after resolution of the cruciform. 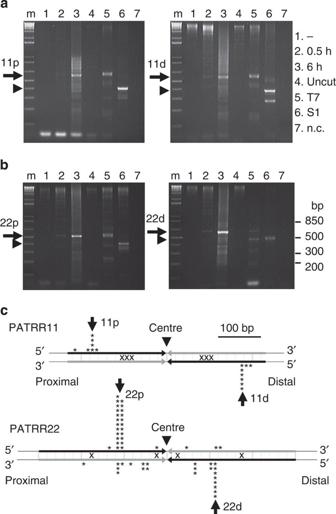Figure 3: Symmetric location of nicks generated by diagonal cleavage of the cruciform-extruding PATRR. (a) 5′ end of DNA breakage on each strand of the PATRR11 plasmid determined by ligation-mediated PCR. The 5′ ends were mapped by PCR in DNA extracted from HEK 293 cells without transfection (lane 1) or obtained at 0.5 (lane 2) or 6 h (lane 3) after transfection with cruciform-extruding P-SD-11. As a size control, a similar PCR reaction was performed on plasmid DNA without treatment (lane 4), treated either with T7 endonuclease I (lane 5) or S1 nuclease (lane 6) and a negative control (n.c.) with no template DNA (lane 7). The size of the major PCR product indicates that the 5′ end of the DNA breaks (thick arrows) are located 180 bp distal to the centre of the PATRR11 (arrowheads) symmetrically on the proximal (left panel, 11p) and distal part (right panel, 11d) of the PATRR. (b) Result of PATRR22 plasmid. The 5′ end of the DNA breaks are located 110 bp distal (arrowheads; 22p and 22d) to the centre of the PATRR22 (arrow). (c) The 5′ ends determined by sequencing of PCR products. Each DNA end is represented by an asterisk. Most of the DNA ends were located at the 5′ portion of the PATRR in each strand (arrowheads). The position of these ends is unrelated to the location of gaps or mismatches between the proximal and distal arms (x). Figure 3: Symmetric location of nicks generated by diagonal cleavage of the cruciform-extruding PATRR. ( a ) 5′ end of DNA breakage on each strand of the PATRR11 plasmid determined by ligation-mediated PCR. The 5′ ends were mapped by PCR in DNA extracted from HEK 293 cells without transfection (lane 1) or obtained at 0.5 (lane 2) or 6 h (lane 3) after transfection with cruciform-extruding P-SD-11. As a size control, a similar PCR reaction was performed on plasmid DNA without treatment (lane 4), treated either with T7 endonuclease I (lane 5) or S1 nuclease (lane 6) and a negative control (n.c.) with no template DNA (lane 7). The size of the major PCR product indicates that the 5′ end of the DNA breaks (thick arrows) are located 180 bp distal to the centre of the PATRR11 (arrowheads) symmetrically on the proximal (left panel, 11p) and distal part (right panel, 11d) of the PATRR. ( b ) Result of PATRR22 plasmid. The 5′ end of the DNA breaks are located 110 bp distal (arrowheads; 22p and 22d) to the centre of the PATRR22 (arrow). ( c ) The 5′ ends determined by sequencing of PCR products. Each DNA end is represented by an asterisk. Most of the DNA ends were located at the 5′ portion of the PATRR in each strand (arrowheads). The position of these ends is unrelated to the location of gaps or mismatches between the proximal and distal arms (x). Full size image Cruciform cleavage is mediated by the Holliday-junction resolvase GEN1 The evidence for diagonal digestion of cruciform DNA suggested that the resolution activity for Holliday-junction structures in mammalian cells [28] could participate in this reaction. MUS81 nuclease, GEN1 and a complex of SLX4-SLX1 have been proposed as candidates for such a resolvase in mammalian cells [29] , [30] , [31] , [32] , [33] , [34] , [35] , [36] , [37] . To identify the cruciform resolvase working in this system, we performed siRNA screening coupled with monitoring the level of diagonal cleavage of the cruciform-extruding plasmids by Southern blot analysis ( Fig. 4a , Supplementary Fig. S3a,b ). Knockdown of GEN1 showed significant reduction of the intensity of the 1.3-kb band corresponding to the cleaved product at the four-way junction in cruciform plasmids. In contrast, knockdown of other candidates, SLX1 and MUS81, did not show significant reduction. The residual cleaved products observed even after the knockdown of GEN1 might possibly be due to the inefficient knockdown of the GEN1 ( Supplementary Fig. S3b ), or redundancy of the resolution activity [38] , [39] , [40] , [41] , [42] . Because functional overlap has been reported between GEN1 and other resolvases, experiments of double knockdown of two of the three enzymes were carried out ( Fig. 4b , Supplementary Fig. S3c,d ). The result of double knockdown of SLX1 and MUS81 did not show any effect. On the other hand, the combination of a GEN1 and SLX1 or a GEN1 and MUS81 knockdown showed a decrease in cleavage similar to that of single knockdown of GEN1 ( Fig. 4a ). These results indicate that the main resolution activity for cruciform cleavage in this system is mediated by GEN1. 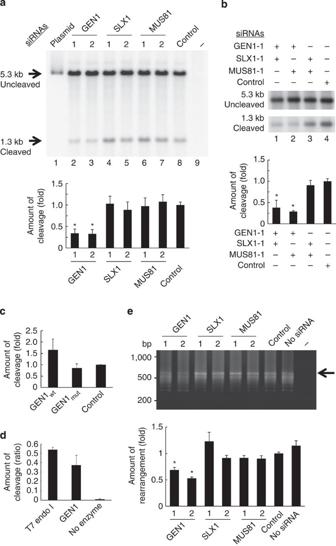Figure 4: Cleavage of the cruciform structure by GEN1. (a) Effect of candidate gene knockdown on cleavage. siRNAs for GEN1, SLX1 or MUS81, as well as control siRNA, were transfected into HEK 293 cells before transfection of a substrate plasmid. After a 3-h transfection of the plasmid, DNAs were collected and subjected to Southern blotting (upper panel), and the cleaved bands were quanrtified relative to the control siRNA (lower panel,n=6). Samples of untransfected plasmid DNA (plasmid) and DNA from untransfected HEK 293 cells (–) were loaded for control. (b) Double knockdown of the combination of the candidate genes. Cleavage was monitored by Southern blot (upper panel) and then quantified (lower panel,n=3). (c) Overexpression of recombinant GEN1 in HEK 293 cells. Only the expression of wild-type GEN1 (GEN1wt) induced the cleavage of the cruciform-extruding plasmid, whereas mutant GEN1 (GEN1mut) or transfection of a control empty vector (control) did not (n=3). (d) Recombinant GEN1 cleaved the PATRR-forming cruciformin vitro. Overexpressed GEN11–527-HIS inE. coliwas purified and used forin vitrocleavage of the PATRR cruciform. Cleavage of the cruciform-extruding plasmid was observed in a way similar to the sample treated with T7 endonuclease I (T7 endo I) (n=3). (e) Translocation-like rearrangement products monitored by semi-quantitative PCR. Decrease of the translocation-like rearrangement molecules (arrow) was observed only in the GEN1 knockdown, which diminished cleavage of the cruciform structure (n=3). Data are presented as means±s.d. Statistical significance against control siRNA was assessed using a Student’st-test: *P<0.01. Figure 4: Cleavage of the cruciform structure by GEN1. ( a ) Effect of candidate gene knockdown on cleavage. siRNAs for GEN1, SLX1 or MUS81, as well as control siRNA, were transfected into HEK 293 cells before transfection of a substrate plasmid. After a 3-h transfection of the plasmid, DNAs were collected and subjected to Southern blotting (upper panel), and the cleaved bands were quanrtified relative to the control siRNA (lower panel, n =6). Samples of untransfected plasmid DNA (plasmid) and DNA from untransfected HEK 293 cells (–) were loaded for control. ( b ) Double knockdown of the combination of the candidate genes. Cleavage was monitored by Southern blot (upper panel) and then quantified (lower panel, n =3). ( c ) Overexpression of recombinant GEN1 in HEK 293 cells. Only the expression of wild-type GEN1 (GEN1 wt ) induced the cleavage of the cruciform-extruding plasmid, whereas mutant GEN1 (GEN1 mut ) or transfection of a control empty vector (control) did not ( n =3). ( d ) Recombinant GEN1 cleaved the PATRR-forming cruciform in vitro . Overexpressed GEN1 1–527 -HIS in E. coli was purified and used for in vitro cleavage of the PATRR cruciform. Cleavage of the cruciform-extruding plasmid was observed in a way similar to the sample treated with T7 endonuclease I (T7 endo I) ( n =3). ( e ) Translocation-like rearrangement products monitored by semi-quantitative PCR. Decrease of the translocation-like rearrangement molecules (arrow) was observed only in the GEN1 knockdown, which diminished cleavage of the cruciform structure ( n =3). Data are presented as means±s.d. Statistical significance against control siRNA was assessed using a Student’s t -test: * P <0.01. Full size image To further support the notion that GEN1 cleaves the cruciform structure of the PATRR plasmids, overexpression of recombinant GEN1 was carried out. Cells that overproduce GEN1 increased the amount of cleaved DNA, but the D157A mutant lacking the nuclease activity did not ( Fig. 4c , Supplementary Fig. S3e ) [31] . When the GEN1 expression vector was transfected into the cells treated with GEN1-siRNA, the GEN1 protein level was restored. The amount of cleaved DNA returned to the level of non-treated cells. However, this effect was not observed when the D157A mutant was transfected ( Supplementary Fig. S3f,g ). In addition, recombinant GEN1 protein purified from Escherichia coli also cut the PATRR-forming cruciform in vitro ( Fig. 4d ). Next, we examined the effect of GEN1 on translocation between the two PATRR plasmids. In our model system, translocation between the two plasmids can fuse a promoter and a green fluorescent protein (GFP) reporter gene, and levels of rearrangement can be estimated by counting GFP-positive cells [19] . We could not detect a significant difference in number of GFP-positive cells possibly because of the low sensitivity of the assay. However, using rearrangement-specific PCR, we confirmed decrease of the translocation-like rearrangement reaction with a knock down of GEN1, but not by a knock down of SLX1 or MUS81 ( Fig. 4e ). These results indicate that both the PATRR11 and PATRR22 plasmids are cleaved at the four-way junction of the cruciform by GEN1, leading to translocations in this model system. Closed hairpin ends are processed by Artemis Based on the results of Southern blot analysis, GEN1 cleaved the cruciform and the DNA ends were converted to a pair of closed hairpin ends. Because translocation breakpoints were located at the centre of the palindromes, a hairpin end is likely opened before fusion with a second DNA end to generate translocation junctions. To identify which hairpin end-specific nucleases participate in translocation formation, we performed siRNA knockdowns in this model system to screen three candidates, Artemis, CtIP and MRE11 ( Supplementary Fig. S4a,b ) [43] , [44] , [45] . Translocation-specific PCR yielded ~650 bp PCR products that correspond to the product from a rearrangement junction derived from a fusion at the centre of the palindromes, similar to the de novo translocations seen in sperm. When Artemis was knocked down, the amount of the ~650 bp major product was greatly reduced ( Fig. 5a ). In contrast, knockdown of CtIP or MRE11 increased the amount of the ~650 bp products. This result suggests that Artemis cleaves at the centre of the hairpin-capped DNA produced by cruciform resolution that leads to the translocation. 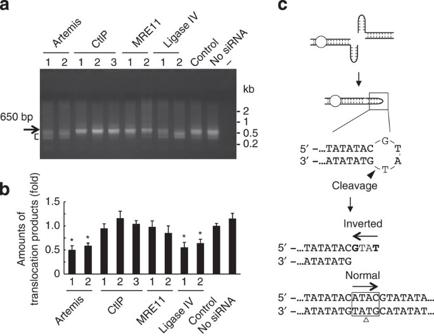Figure 5: Artemis cleaves newly formed hairpin ends. (a) Rearrangement-specific PCR of the samples obtained after knockdown of candidate genes. Several siRNAs for Artemis, CtIP, MRE11 or ligase IV, as well as a control siRNA, were transfected into HEK 293 cells before the transfection of substrate plasmids. At 24 h after transfection of the plasmids, the DNAs were collected and translocation-specific PCR was carried out (left). The top band at ~650 bp (an arrow) corresponds to a product derived from fusion at the tips of the hairpins of PATRR11 and 22. Knockdown of Artemis and ligase IV specifically reduced the top band, indicating that these enzymes were involved in generation of the translocation. Some minor bands below the top band (bracket) were by-products of the model system, because these shorter products cannot be observed when the same translocation-specific PCR was performed to detectde novotranslocations in sperm samples from human males. (b) Quantification of the ~650 bp PCR products (n=3). (c) Schematic representation of the central inversion produced by Artemis cleavage at 2 bp distal from the tip of the hairpin. Data are presented as means±s.d. Statistical significance against control siRNA was assessed using a Student’st-test: *P<0.01. Figure 5: Artemis cleaves newly formed hairpin ends. ( a ) Rearrangement-specific PCR of the samples obtained after knockdown of candidate genes. Several siRNAs for Artemis, CtIP, MRE11 or ligase IV, as well as a control siRNA, were transfected into HEK 293 cells before the transfection of substrate plasmids. At 24 h after transfection of the plasmids, the DNAs were collected and translocation-specific PCR was carried out (left). The top band at ~650 bp (an arrow) corresponds to a product derived from fusion at the tips of the hairpins of PATRR11 and 22. Knockdown of Artemis and ligase IV specifically reduced the top band, indicating that these enzymes were involved in generation of the translocation. Some minor bands below the top band (bracket) were by-products of the model system, because these shorter products cannot be observed when the same translocation-specific PCR was performed to detect de novo translocations in sperm samples from human males. ( b ) Quantification of the ~650 bp PCR products ( n =3). ( c ) Schematic representation of the central inversion produced by Artemis cleavage at 2 bp distal from the tip of the hairpin. Data are presented as means±s.d. Statistical significance against control siRNA was assessed using a Student’s t -test: * P <0.01. Full size image Artemis has been reported to cleave hairpin ends, making a two-nucleotide overhang at the 3′ end [43] . This may produce an inversion at the central four nucleotides of the palindrome in junction sequences of the translocation ( Fig. 5c ). This phenomenon is evidenced by nucleotide differences between the proximal and distal arms, one nucleotide downstream of centre. A total of 14 junction sequences that escaped central deletion and retained the palindromic centre could be analysed. An ‘A’ that was originally located on the proximal arm was replaced by a ‘G’ on the distal arm in seven translocation junctions. This proximal-to-distal exchange in the central region may also indicate diagonal cutting of the cruciform similar to that seen in the arm. However, proximal-to-distal substitution at the central region appears to occur independently of that in the arm region. This small inversion at the centre is similar to P nucleotides introduced at the junction of V(D)J recombination, in which Artemis participates in the hairpin opening of intermediate products [46] . These data lend support to the idea that hairpin-capped DNA produced by cleavage of the four-way cruciform junction by GEN1 undergoes a second cleavage at the hairpin tip by Artemis. The junction sequence derived from the model system indicates NHEJ, in which three quarters of junctions had microhomologies of less than four nucleotides [19] . To confirm that the final joining reaction was performed by ligase IV, we knocked down ligase IV using siRNA ( Fig. 5a , Supplementary Fig. S4c ). PCR products from the translocation junction are decreased, indicating involvement of ligase IV in the final step of translocation formation. Thus, the rejoining of opened hairpin DNA ends were carried out by NHEJ, possibly using the same machinery as the later reaction of V(D)J recombination [47] , [48] , [49] . Evidence of cruciform resolution in sperm Assuming that the PATRRs on human chromosomes 11 and 22 are actually cut diagonally at the four-way junction of extruded cruciforms during formation of the t (11;22), sequence exchange between the proximal and distal arms seen in this plasmid system should also be observed in actual t (11;22)s in humans. We examined a total of 144 de novo translocation products in sperm from a single individual who carries nucleotide differences that allow one to distinguish between the proximal and distal arms of PATRR11. We detected 11 translocations (7.6%) with evidence for proximal-to-distal exchanges. In the PATRR22 region, 5 out of 54 (9.3%) translocations indicated proximal-to-distal exchange. The presence of the exchanges strongly suggests that cruciform resolution actually takes place in the process of t (11;22) development in spermatogenesis. Although the proportion of translocations with the exchange was less than that seen in the plasmid model system, we speculate that this difference is explained by the preference of the nicked strand as a target for MMR [50] , [51] . After the PATRR is cut diagonally at the cruciform four-way junction, newly formed hairpin-capped DNA ends should carry nicks on either strand. It is possible that the repair system preferentially corrects the mismatch on the nicked strand using the intact strand as a template, resulting in template bias. In case of the plasmid system, most of the nicks appear to be repaired immediately after cleavage, resulting in equivalent usage of both strands as templates. In addition, proximal-to-distal exchange was also observed at the centre of the palindrome of de novo t (11;22) junctions in human sperm. In five junction sequences that escaped central deletion and retain their palindromic centre, two manifested the exchange pattern at the centre without exchanges in the arm, whereas the other two had no central exchange with proximal-to-distal exchanges in the arm. These data suggest that exchanges in the centre are independent of those in palindromic arms. These findings are similar to what was observed in the plasmid model system. It is likely that Artemis also cleaves hairpin ends produced by cruciform resolution in the process of de novo translocation formation in sperm, introducing additional proximal-to-distal exchanges near the translocation junction. Therefore, based on the presence of both types of proximal-to-distal exchange in the junction fragment sequences of de novo t (11;22)s in sperm DNA, we conclude that the PATRR adopts unusual cruciform structures in spermatogenic cells, and that a diagonal cut at the four-way junction of the cruciform followed by opening of the hairpin-capped DNA ends leads to the recurrent chromosomal translocation in humans ( Fig. 6 ). 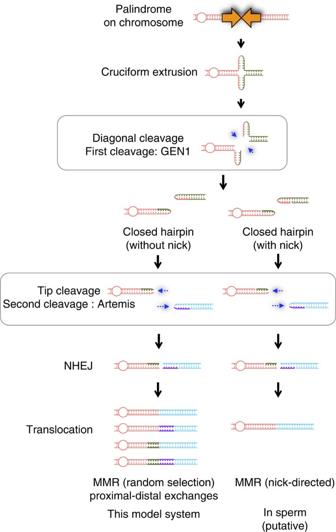Figure 6: Model of palindrome-mediated translocation in humans. Cruciform extrusion leads to the sequential cleavage by GEN1 and Artemis. The diagonal cleavage produces a nick at the base of the cruciform, which is sealed by intrinsic ligase activity in the model system. The resulting closed hairpin leads to random selection of the template strand for MMR, manifesting frequent proximal–distal exchanges at the junction of the rearranged molecules. In contrast, a hairpin with a residual nick at the base of the cruciform could produce a bias in template-strand selection for the MMR reaction, resulting in a lower incidence of proximal–distal exchanges at the junction ofde novotranslocations in sperm. Figure 6: Model of palindrome-mediated translocation in humans. Cruciform extrusion leads to the sequential cleavage by GEN1 and Artemis. The diagonal cleavage produces a nick at the base of the cruciform, which is sealed by intrinsic ligase activity in the model system. The resulting closed hairpin leads to random selection of the template strand for MMR, manifesting frequent proximal–distal exchanges at the junction of the rearranged molecules. In contrast, a hairpin with a residual nick at the base of the cruciform could produce a bias in template-strand selection for the MMR reaction, resulting in a lower incidence of proximal–distal exchanges at the junction of de novo translocations in sperm. Full size image In this report we propose a ‘two-step hypothesis’ for the generation of PATRR-mediated translocations. GEN1 and Artemis, which normally work independently in the homologous recombination and NHEJ pathways, appear to have a crucial role in the development of palindrome-mediated translocations in our model system. Indeed, depletion of Holliday-junction resolvases induces chromosome instability, and defects in Artemis induce increased cellular radiosensitivity [42] , [52] . However, the emergence of unusual DNA structures at palindromic DNA in certain conditions triggers successive misrecognition of the substrate by GEN1 and Artemis. These two independent pathways may act in concert on the unusual secondary structure, resulting in the recurrent GCR or genomic instability in the human genome. Besides the recurrent constitutional t (11;22), several recurrent and non-recurrent chromosomal translocations in humans have been reported to be mediated by palindromic DNA. This report proposes a common pathway leading to these palindrome-mediated translocations in humans. Previously, a ‘centre-break mechanism’ of cruciform disruption had been proposed for palindrome-mediated rearrangements. In this study, rearrangement junctions carry small central deletions, suggesting ‘centre breakage’. However, we demonstrated (1) the presence of hairpin-capped DNA ends by Southern analyses, (2) residual nicks that indicate diagonal cleavage, (3) proximal-to-distal nucleotide exchanges at the palindromic arm sequence of the translocation junction and (4) the presence of heteroduplex DNA in the translocation junction after inhibition of MMR. All of this evidence lend support to a mechanism involving resolution of the four-way junction of a cruciform structure. Data from siRNA experiments showed that GEN1, a Holliday-junction resolvase, participates in the first step in the development of palindrome-mediated translocations. The initial cleaved product was closed hairpin-ended DNA, which suggests that diagonal cleavage produces ligase-sensitive nicks. In addition, we detected symmetrically cleaved DNA ends by means of ligation-mediated PCR, which support the involvement of GEN1 (ref. 31 ). However, another candidate MUS81-EME1 cuts the asymmetrical sites of synthetic Holliday junctions on strands of similar polarity, making ligase-resistant nicks [29] . The other candidate SLX1-SLX4 complex would cut symmetric sites at the four-way junction [33] , [34] , [35] . Our siRNA experiments do not support the participation of MUS81-EME1 nor SLX1-SLX4 in the development of the translocation. Despite of the functional redundancy, it is still unclear why GEN1 prefers to resolve the cruciform of the PATRR in this model system. Specificities of structure, for example, cruciform size or nucleotide sequence near the four-way junction, might affect such preferences. Data from siRNA experiments show that Artemis participates in the second cleavage to open the tip of the closed hairpin ends produced by GEN1. Endonuclease activity of Artemis requires binding to the DNA-activated DNA-PKcs, followed by phosphorylation by DNA-PKcs with broken DNA ends [53] . It has been reported that the presence of hairpin-ended DNA will stimulate activation of the Artemis:DNA-PKcs complex to produce a nick at the hairpin tip [54] . A final step is NHEJ that leads to illegitimate chromosomal rejoining by ligase IV. These reactions appear to be similar to coding joint formation in the V(D)J recombination reaction. It is conceivable that a certain pathway might be involved in the reaction, bringing two hairpin-capped DNA ends on different chromosomes into close proximity to produce translocations between palindromes, like coding joint formation. Finally, we found evidence of the ‘two-step cleavage’ mechanism in de novo translocation junctions in sperm from normal males. Both GEN1 and Artemis have crucial functions in the DNA-repair machinery, acting ubiquitously in a variety of cell types including testis [52] . Because de novo t (11;22)s have been detected only in sperm, we speculate that cruciform formation at the PATRR only takes place during spermatogenesis [22] . One possibility that can explain this sperm specificity is the high number of DNA replications. Indeed, cruciform extrusion and replication stalling at palindromic regions have been demonstrated in yeast [7] , [55] . However, the translocation is completely recapitulated in the model system using non-replicating plasmids, which implies a mechanism that does not rely on DNA replication: perhaps a post-meiosis hypothesis [8] . In the late stage of spermatogenesis, a transition of DNA from histone to protamine takes place, providing the opportunity for dynamic changes of DNA conformation. Because removal of a single nucleosome structure induces one negative supercoil [56] , the accumulation of local negative supercoiling during the histone-protamine transition period could induce an unusual cruciform conformation of the palindrome. Such massive histone removal may not occur in somatic cells, which could explain the sperm-specific development of t (11;22)s. In mice, round spermatids were shown to have NHEJ activity [57] . On the other hand, a recent finding suggests that GEN1 acts in meiosis II, but it is still unclear whether the GEN1 also acts in post-meiotic cells or not [58] . A more thorough investigation using model animals might reinforce the post-meiosis hypothesis. Plasmid DNAs, siRNAs and primers Plasmid construction of the translocation model system (P-SD-11 and 22-SA-GFP) and preparation of cruciform-extruding or -unextruding plasmids by using alkaline-SDS method or Triton method, respectively [19] . In brief, bacteria were lysed by alkaline or 3% Triton X-100 solutions followed by column purification at 4 °C. For siRNA experiments, the plasmids were further purified by CsCl density gradient ultracentrifugation. The siRNAs for the candidate genes ( Supplementary Table S3 ) and a control (12935-110) were purchased from Invitrogen. Primers used for PCR and cloning were shown in Supplementary Table S4 . Transfection For siRNA transfection, HEK 293 cells were seeded at 5 × 10 4 cell per ml in 30 mm dishes. After 24 h, siRNAs were transfected at 40 nM using Lipofectamine RNAiMax (Invitrogen). Additional siRNA transfection was carried out to accomplish knockdown of GEN1 , SLX1 and MUS81 genes at 80 nM 36 h after the first transfection. After 36 h of siRNA transfection, the medium was changed, and a total of 3.2 μg of plasmid DNA was transfected using Lipofectamine 2000 (Invitrogen). The reaction was stopped after 1–2 h by changing the medium. Sample preparation for DNAs, RNAs and proteins The cells were detached from the dishes by pipetting, divided into tubes and washed twice with PBS. DNAs were purified using DNAzol (Cosmo Bio) after additional wash with PBS to remove untransfected DNAs. RNAs were purified using FastPure RNA Kit (Takara Bio). For western blotting, the cells were resuspended in PBS, lysed by adding an equal volume of 2 × sample buffer (0.125 M Tris-Cl, pH 6.8, 4% SDS, 10% sucrose, 10% 2-mercaptoethanol and 0.004% bromophenol blue) and boiled for 6 min. Detection of DNA rearrangement in HEK 293 cells Semi-quantitative PCR from 100 ng of purified DNA was carried out for the detection of the rearrangement in transfected cells. The PCR conditions were 25 cycles of 10 s at 98 °C and 5 min at 60 °C [19] . For single-molecule PCR, DNA was diluted and 25 pg was used for each reaction. We carried out extended cycles (40 cycles) of PCR and obtained 36 products from 192 wells. The products were isolated and subjected to direct sequencing. The products showing heterologous sequence were cloned into pT7Blue T-vector (Novagen), and the sequences of both molecules were determined. We excluded the products containing more than a single rearranged molecule, which were judged by exhibiting different breakpoints among the molecules. Detection of the 5′ ends of transfected DNAs by ligation-mediated PCR DNAs from cells at 0.5 and 6 h after transfection were subjected to double-stranded DNA synthesis from first strand primers, generating a blunt end at the breakage site [59] . After ligating a double-stranded linker, 30 cycles of PCR were carried out using PATRR-optimized conditions [27] , which is at 98 °C for 10 s and at 60 °C for 5 min. For size controls, plasmids with extruded PATRRs were treated with T7 endonuclease I or S1 nuclease and similarly used as PCR template. Detection of gene expression Expression level of each gene was quantified by quantitative PCR with reverse transcription. An amount of 1 μg of total RNA was reverse transcribed by using Primescript RT Master Mix (Takara Bio), and real-time PCR was carried out by using SYBR Premix Ex Taq II (Takara Bio) and 7300 Real-time PCR system (Applied Biosystems). HPRT gene was used for internal control. Primers were shown below. An antibody for human GEN1 was a gift from Dr Stephen C. West. Other antibodies for human MUS81 (MTA30; ImmuQuest), Artemis (PAB-10241; Orbigen), MRE11 (12D7; GeneTex), GAPDH (6C5; Chemicon International), TP53 (PAb 240; BD Pharmingen) and GFP (598; MBL) were purchased from the manufacturers. Recombinant GEN1 expression For transfection to HEK 293 cells, an overexpression vector of wild-type GEN1 was constructed by cloning of human full-length GEN1 into a modified pIRES2-EGFP vector (Clontech), promoter of which was substituted with the promoter and intron part of CAGGS expression vector [60] by digesting with Ase I and Nhe I (CAG-IRES2-GEN1-EGFP). PCR with reverse transcription was carried out from HEK 293 RNA. After cloning of the PCR product digested with Xho I and Bam HI, nucleotide sequence of the clone was confirmed that it had no coding change compared with that in the database. A mutant GEN1 (D157A) [31] vector was produced by modifying the vector of wild-type GEN1 using Primestar Mutagenesis Kit (Takara Bio). These two vectors as well as an empty vector were transfected into HEK 293 cells, and the plasmids for translocation model system were transfected after 48 h. For restoration assay of knockdown GEN1 by transient expression vector, pACYC184 plasmid DNA was added for adjusting the DNA amount of transfection. For in vitro cleavage of PATRR cruciforms, an N-terminal fragment of GEN1, GEN1 1–527 -HIS, which had been shown to be an active form [31] , was constructed by amplifying corresponding region of human GEN1 from HEK 293 RNA. The product was cloned into pET-32b vector (Novagen) that has been removed N-terminal tags by digesting Nde I and Xho I (pET-GEN1-HIS). The construct was transfected into E. coli BL21(DE3) (Invitrogen) and cultured in Luria broth until OD 600 reached to 0.5. Induction of the protein expression was carried out by 0.1 mM IPTG for overnight at 16 °C. The cell was collected and solubilized by sonication in a buffer (300 mM NaCl and 50 mM NaH 2 PO 4 , pH 8.0) at 0 °C, and the soluble part was loaded onto Ni-NTA spin column (Qiagen). After washing the column three times with the buffers supplemented with 20 and 100 mM imidazole, respectively, GEN1 was eluted in the buffer with 500 mM imidazole. About 5 ng of the eluted protein was used for digestion of the cruciform structure in a reaction buffer (10 mM Tris-acetate, pH 7.4, 50 mM potassium acetate, 5 mM magnesium acetate, 1.0 mM dithiothreitol and 0.01% BSA) at 25 °C for 15 min. For a positive control, 5 U of T7 endonuclease I (NEB) was used following the manufacturer’s instruction. Detection of the t (11;22) in sperm About 2–5 × 10 7 sperm was collected from semen with wash twice by PBS, and the DNA was purified by Puregene DNA isolation Kit (Gentra) with adding 50 mM dithiothreitol during lysis step according to the manufacturer’s instruction. The quality and quantity of the resulting high-molecular weight DNA (>10 kb, 50–100 μg) was determined by both ultraviolet spectrophotometry and agarose gel electrophoresis. De novo translocations of t (11;22) in human sperm were detected by single-molecule PCR as described above. For this sperm sample, 10 ng of template DNA was suitable for separation of each junction product [11] . Accession code: OMIM no. 609029. How to cite this article: Inagaki, H. et al. Two sequential cleavage reactions on cruciform DNA structures cause palindrome-mediated chromosomal translocations. Nat. Commun. 4:1592 doi: 10.1038/ncomms2595 (2013).